Intestinal stem cells lacking the Math1 tumour suppressor are refractory to Notch inhibitors Intestinal cells are constantly produced from a stem cell reservoir that gives rise to proliferating transient amplifying cells, which subsequently differentiate into one of the four principal cell types. Signalling pathways, including the Notch signalling pathway, coordinate these differentiation processes and their deregulation may cause cancer. Pharmacological inhibition through γ-secretase inhibitors or genetic inactivation of the Notch signalling pathway results in the complete loss of proliferating crypt progenitors due to their conversion into post-mitotic goblet cells. The basic helix–loop–helix transcription factor Math1 is essential for intestinal secretory cell differentiation. Because of the critical roles of both Math1 and Notch signalling in intestinal homeostasis and neoplastic transformation, we sought to determine the genetic hierarchy regulating the differentiation of intestinal stem cells into secretory cells. In this paper, we demonstrate that the conversion of intestinal stem cells into goblet cells upon inhibition of the Notch signalling pathway requires Math1. The intestine is a self-renewing tissue with a high turnover rate in which a specialized epithelium performs its primary functions of digestion, absorption, protection and excretion. The small intestinal epithelium consists of a proliferative compartment (the crypt of Lieberkühn) and a differentiated, functional compartment (the villus). The continuously produced new intestinal epithelial cells are derived from leucine-rich repeat-containing G-protein-coupled receptor 5 (Lgr5) and olfactomedin-4 (Olfm4)-expressing multipotent stem cells, also known as crypt base columnar cells (CBC's) [1] , [2] . In addition to supporting normal epithelial homeostasis, intestinal stem cells are considered to have an important role in tissue regeneration and, upon introduction of certain mutations, they serve as the cells-of-origin of intestinal cancer [3] . Each crypt contains at least six long-lived stem cells that are not quiescent, but divide every day [1] . They give rise to the so-called transit-amplifying cells that reside in the crypt and migrate along the crypt–villus axis. During migration, intestinal epithelial cells exit the mitotic cell cycle and differentiate into one of the four principal cell types: mucus-secreting goblet cells, hormone-secreting enteroendocrine cells, antimicrobial peptide-secreting Paneth cells and hydrolase-secreting enterocytes. Enterocytes, goblet and enteroendocrine cells continue migrating up the villus, whereas Paneth cells migrate downwards to reside at the crypt base [4] . The basic helix–loop–helix transcription factor Math1 is important for cell fate determination in multiple tissues. Math1-null embryos die at birth because of respiratory failure and lack many specific cell lineages, including cerebellar granule neurons, spinal cord interneurons and inner ear hair cells [5] , [6] , [7] . Moreover, the intestines of Math1-deficient neonatal mice show a relatively normal crypt-villus architecture that is populated entirely by enterocytes, indicating that Math1 is required for all secretory cell lineages. Deletion of Math1 in the adult intestine also results in the loss of all secretory cells, indicating a similar role in intestinal homeostasis [8] . More recently, Math1 was shown to have a tumour suppressor function in colorectal neoplasia and its function is lost in some patients with colorectal cancer [9] . The Notch pathway shapes cellular repertoires in a variety of embryonic tissues by inducing or inhibiting cell fate commitment in a context-dependent manner. The best-characterized Notch target genes are the basic helix–loop–helix proteins hairy/enhancer of split. These proteins repress the expression of epithelial cell fate determination genes such as neurogenin ( ngn ), Achaete-Scute and Math1 [10] . Genetic loss-of-function experiments in mice show that Notch signalling regulates a binary cell fate decision of intestinal progenitors between secretory and absorptive lineages [11] . Furthermore, conditional gut-specific inactivation of RBP-J, which mediates signalling by all four Notch receptors, results in the complete loss of proliferating crypt progenitors and conversion into post-mitotic goblet cells [12] . Conversely, transgenic expression of the Notch intracellular domain yields the reciprocal phenotypes and results in a block of secretory cell differentiation and expansion of immature progenitors [13] . Additional support for the control of intestinal cell fate by Notch stems from the use of γ-secretase inhibitors (GSIs), which block the generation of Notch intracellular domain. Rodents treated with GSI dibenzazepine (DBZ) display a huge increase in goblet cell numbers in the gut, completely mimicking the phenotype of RBP-J mice in this respect [12] . These studies indicate an essential role for Notch signalling as a gatekeeper of the gut progenitor compartment. Moreover, DBZ also induces goblet cell differentiation in adenomas of mice carrying a mutation in the Apc tumour suppressor gene. This has led to the idea that GSIs, originally developed for the treatment of Alzheimer's disease, might be of therapeutic benefit in colorectal neoplastic disease [12] , [14] . Because of the critical roles of both Math1 and Notch signalling in intestinal homeostasis and neoplastic transformation, we sought to determine the genetic hierarchy regulating the differentiation of intestinal stem cells into secretory cells. To this end, we compared the effects of the loss of Math1 alone, Notch signalling alone or both on mouse adult intestinal (stem) cell conversion. Here, we demonstrate that the conversion of intestinal stem cells into goblet cells after inhibition of the Notch signalling pathway requires Math1. Absence of the secretory lineage upon removal of Math1 To determine the role of Math1 in intestinal homeostasis, we generated a compound mouse from floxed Math1 and AHCre mice. AHCre mice carry the Cre enzyme under the control of the inducible Cyp1A promoter [15] . After intraperitoneal (IP) injection of β-naphthoflavone, this cre allele is activated in several internal organs, including the epithelium of the small intestine, thereby deleting the floxed Math1 allele ( Fig. 1a,b ). Analysis of the intestine, using cell type-specific reagents against goblet cells ( Fig. 1c,d ; Periodic acid-Schiff (PAS) staining), enteroendocrine cells ( Fig. 1e,f ; synaptophysin staining) and Paneth cells ( Fig. 1g,h ; lysozyme staining), showed an almost complete absence of the secretory lineage (goblet cells, Paneth cells and enteroendocrine cells), but not the enterocyte lineage ( Fig. 1i,j ; alkaline phosphatase staining), on deletion of Math1. However, staining for the proliferation marker Ki67 ( Fig. 1k,l ) showed that crypt cells still proliferate. Therefore, Math1 is essential for adult intestinal secretory cell production, but is not required for proliferating progenitor cells. These results confirm and extend previous analysis of the Math1-deficient intestine using floxed Math1 mice crossed with Fabpl 4XAT_132 Cre transgenic mice that express Cre in a mosaic pattern in the distal intestine and colon, but not in the jejunum and proximal ileum [8] . 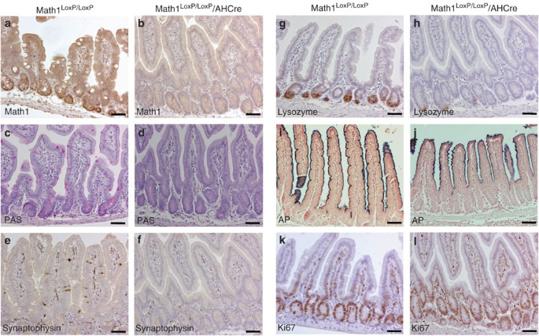Figure 1: Absence of the intestinal secretory lineage on removal of the transcription factor Math1. Immunohistochemical analysis of the small intestine from Math1LoxP/LoxP/AHCre mice (b,d,f,h,j,l) and control Math1LoxP/LoxPmice (a,c,e,g,i,k) after deletion of Math1 on induction of the Cre enzyme with β-naphthoflavone, if applicable. The absence of Math1 after Cre induction was confirmed by staining for Math1 protein (bversusa), the absence of goblet cells is shown by Periodic acid-Schiff staining (PAS) (dversusc), absence of enteroendocrine cells is shown by synaptophysin staining (fversuse), the strong reduction of Paneth cells is shown by lysozyme staining (hversusg) and the presence of enterocytes by alkaline phosphatase (AP) staining (jversusi). Staining for proliferation marker Ki67 (lversusk) showed that cell proliferation had not changed. Scale bar is 100 μm. Figure 1: Absence of the intestinal secretory lineage on removal of the transcription factor Math1. Immunohistochemical analysis of the small intestine from Math1 LoxP/LoxP /AHCre mice ( b , d , f , h , j , l ) and control Math1 LoxP/LoxP mice ( a , c , e , g , i , k ) after deletion of Math1 on induction of the Cre enzyme with β-naphthoflavone, if applicable. The absence of Math1 after Cre induction was confirmed by staining for Math1 protein ( b versus a ), the absence of goblet cells is shown by Periodic acid-Schiff staining (PAS) ( d versus c ), absence of enteroendocrine cells is shown by synaptophysin staining ( f versus e ), the strong reduction of Paneth cells is shown by lysozyme staining ( h versus g ) and the presence of enterocytes by alkaline phosphatase (AP) staining ( j versus i ). Staining for proliferation marker Ki67 ( l versus k ) showed that cell proliferation had not changed. Scale bar is 100 μm. Full size image Math1 is required for goblet cell conversion We next investigated the consequence of Math1 deletion, followed by inhibition of the Notch signalling pathway, on intestinal homeostasis. Math1 LoxP/LoxP mice were used as genetic background controls for the stainings ( Fig. 2a–e ). To examine the effect of loss of Notch signalling, we used Math1 LoxP/LoxP mice without AHCre, which were treated with GSI DBZ ( Fig. 2f–j ). As expected [12] , inhibition of Notch signalling in the intestine of Math1 LoxP/LoxP mice results in the following: a massive conversion of cells into PAS + goblet cells ( Fig. 2f ), the presence of lysozyme + Paneth cells ( Fig. 2g ), a complete block of epithelial cell division as shown by staining for the proliferation marker Ki67 ( Fig. 2h ), the induction of the Math1 protein ( Fig. 2i ) and loss of the Notch1 effector Hes1 ( Fig. 2j ). This phenotype was exactly the same in the control heterozygous Math1/AH-cre or AH-cre mice. GSI-induced Notch inhibition in the intestine of mice in which Math1 had been deleted (Math1 LoxP/LoxP /AHCre) shows the absolute requirement of Math1 for this phenotype. These mice show an almost complete absence of secretory lineage in the crypts in which Math1 was successfully deleted. Specifically, we observe the lack of goblet cells ( Fig. 2k ), a strong reduction of Paneth cells ( Fig. 2l ), the presence of normal cell proliferation ( Fig. 2m ), the absence of the Math1 protein ( Fig. 2n ) and the absence of the Notch effector Hes1 ( Fig. 2o ). Internal control crypts in which Math1 was not deleted (box in Fig. 2n ) show that GSI treatment worked because these crypts show goblet cell conversion (box in Fig. 2k ) and a robust block of cell proliferation (box in Fig. 2m ). Therefore, Math1 is required for the induction of secretory cell fate on disruption of Notch signalling. 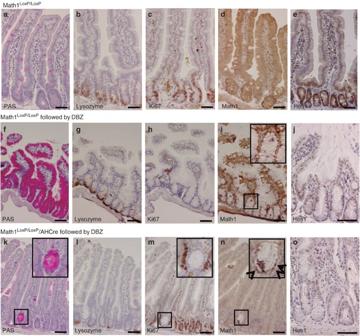Figure 2: Math1 is required for goblet cell conversion downstream of the Notch signalling pathway. Immunohistochemical analysis of the small intestine from Math1LoxP/LoxPmice as genetic background controls for the stainings (a–e) and that from Math1LoxP/LoxPmice after treatment with the gamma secretase inhibitor dibenzazepine (DBZ) (f–j) and Math1LoxP/LoxP/AHCre mice (k–o) after deletion of Math1 on the induction of the Cre enzyme with β-naphthoflavone, followed by disruption of the Notch signalling pathway using DBZ. Goblet cells are stained by a Periodic acid-Schiff staining (PAS) (a,f,k), Paneth cells by an antibody directed against lysozyme (b,g,l), proliferating cells by an antibody directed against Ki67 (c,h,m), Math1 (d,i,n) and Hes1 (e,j,o) by an antibody directed against Math1 and Hes1, respectively. The mice have been correctly treated with DBZ as the crypt that did not undergo Math1 deletion (box inn, arrows indicate Math1-positive cells) showed goblet cell conversion (box ink) and block of cell proliferation (box inm). Scale bar is 100 μm. Figure 2: Math1 is required for goblet cell conversion downstream of the Notch signalling pathway. Immunohistochemical analysis of the small intestine from Math1 LoxP/LoxP mice as genetic background controls for the stainings ( a – e ) and that from Math1 LoxP/LoxP mice after treatment with the gamma secretase inhibitor dibenzazepine (DBZ) ( f – j ) and Math1 LoxP/LoxP /AHCre mice ( k – o ) after deletion of Math1 on the induction of the Cre enzyme with β-naphthoflavone, followed by disruption of the Notch signalling pathway using DBZ. Goblet cells are stained by a Periodic acid-Schiff staining (PAS) ( a , f , k ), Paneth cells by an antibody directed against lysozyme ( b , g , l ), proliferating cells by an antibody directed against Ki67 ( c , h , m ), Math1 ( d , i , n ) and Hes1 ( e , j , o ) by an antibody directed against Math1 and Hes1, respectively. The mice have been correctly treated with DBZ as the crypt that did not undergo Math1 deletion (box in n , arrows indicate Math1-positive cells) showed goblet cell conversion (box in k ) and block of cell proliferation (box in m ). Scale bar is 100 μm. Full size image Goblet cell conversion of stem cells requires Math1 To determine whether the antagonistic interactions between Math1 and Notch signalling affect intestinal stem cells, we investigated the consequence of Math1 deletion combined with Notch inhibition on this compartment. Olfm4 is a well-documented specific marker of mouse and human intestinal stem cells [2] , [16] . We therefore analysed the intestines derived from Math1 LoxP/LoxP control mice ( Fig. 3a ), Math1 LoxP/LoxP /AHCre mice on Cre induction ( Fig. 3b ), Math1 LoxP/LoxP mice treated with DBZ ( Fig. 3c ) and Math1 LoxP/LoxP /AHCre mice on Cre induction followed by DBZ treatment ( Fig. 3d ) for the presence or absence of stem cells using Olfm4 in situ hybridization combined with the presence or absence of goblet cells using PAS staining. The analysis of the intestine of Math1 LoxP/LoxP control mice shows the presence of normal numbers of Olfm4 + intestinal stem cells at the bottom of crypts and normal numbers of PAS + goblet cells ( Fig. 3a ). The analysis of the intestine of Math1 LoxP/LoxP /AHCre mice following Cre induction with β-naphthoflavone shows the presence of normal numbers of Olfm4 + stem cells at the bottom of the crypts, but an absence of PAS + goblet cells ( Fig. 3b ). These data suggest that intestinal stem cells do not require Math1. The analysis of the intestine of Math1 LoxP/LoxP mice after disruption of the Notch signalling pathway using GSI DBZ ( Fig. 3c ) shows a complete absence of Olfm4 + stem cells and the concomitant appearance of PAS + goblet cells in the stem cell zone. These data imply that all intestinal stem cells are converted into goblet cells on inhibition of the Notch signalling pathway. In contrast, the analysis of the intestine of Math1 LoxP/LoxP /AHCre mice after Math1 deletion, followed by disruption of the Notch signalling pathway by DBZ, shows the presence of normal numbers of Olfm4 + stem cells and the absence of PAS-staining goblet cells ( Fig. 3d ). Therefore, Math1 is required for the conversion of intestinal stem cells on inhibition of the Notch signalling pathway. 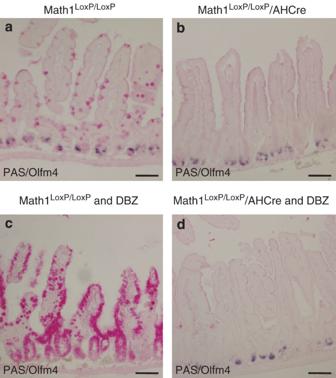Figure 3: Math1 is required for the differentiation of intestinal stem cells into goblet cells on Notch signalling inhibition. Immunohistochemical analysis of small intestine from Math1LoxP/LoxP(a), Math1LoxP/LoxP/AHCre mice after deletion of Math1 (b), Math1LoxP/LoxPtreated with dibenzazepine (DBZ) (30 μmol kg−1) to block the Notch pathway (c) and Math1LoxP/LoxP/AHCre mice after deletion of Math1 on induction of the Cre enzyme, followed by pharmacological disruption of the Notch signalling pathway using DBZ (d) with the intestinal stem cell-specific marker Olmf4 (blue), in combination with a PAS staining (magenta) for goblet cells. Scale bar is 100 μm. Figure 3: Math1 is required for the differentiation of intestinal stem cells into goblet cells on Notch signalling inhibition. Immunohistochemical analysis of small intestine from Math1 LoxP/LoxP ( a ), Math1 LoxP/LoxP /AHCre mice after deletion of Math1 ( b ), Math1 LoxP/LoxP treated with dibenzazepine (DBZ) (30 μmol kg −1 ) to block the Notch pathway ( c ) and Math1 LoxP/LoxP /AHCre mice after deletion of Math1 on induction of the Cre enzyme, followed by pharmacological disruption of the Notch signalling pathway using DBZ ( d ) with the intestinal stem cell-specific marker Olmf4 (blue), in combination with a PAS staining (magenta) for goblet cells. Scale bar is 100 μm. Full size image In conclusion, these data demonstrate that Math1 is essential for the differentiation of intestinal stem cells induced by inhibition of the Notch signalling pathway, and that therefore Math1 functions downstream of Notch signalling to induce cell cycle exit and differentiation in the intestinal epithelium. This suggests that under normal conditions Notch signalling is required to maintain stem cells in an uncommitted state until Math1 is activated. Our data have potential implications for intestinal tumours as well. We recently proposed that inhibition of the Notch pathway might provide an alternative targeted-drug strategy for the treatment of colorectal neoplasia by converting adenomas in mice into post-mitotic goblet cells [12] . However, we also showed that Math1 functions as a tumour suppressor gene in colorectal cancer, and may be lost in a number of primary human tumours [9] . The current study shows that Notch inhibition may only be a useful therapy for intestinal tumours if Math1 function is intact or if it can be induced. An active population of Math1 mutant stem cells may give rise to tumours either because of loss of capacity to differentiate or because of the specific absence of goblet cells that secrete the mucus barrier. Goblet cells are known to be depleted in mucin-depleted foci that are considered to be direct precursors of intestinal tumours. In support of this idea, ablation of mucin leads to tumour formation even without loss of differentiation [17] , [18] , [19] , [20] . Generation of Math1 LoxP/LoxP /AHCre The transgenic line AHCre [15] was crossed with LoxP Math1 mice (generated and kindly provided by Dr Huda Zoghbi, Baylor College of Medicine, Houston, TX, USA) to obtain Math1 LoxP/LoxP /AHCre mice, as well as various genotypic controls. The Cre enzyme was induced by a single IP injection of 200 μl of β-naphthoflavone (10 mg ml −1 ; Sigma Aldrich) dissolved in corn oil on day 0. The mice were killed on day 14. All procedures were performed in compliance with local animal welfare laws, guidelines and policies. Treatment of animals with the γ-secretase inhibitor DBZ Dibenzazepine (3 g) was custom synthesized to more than 99.9% purity by Syncom (Groningen, The Netherlands). DBZ was suspended finely in 0.5% (w/v) hydroxypropylmethylcellulose (Methocel E4M) and 0.1% (w/v) Tween 80 in water. The Notch signalling pathway was blocked by a single IP injection of GSI DBZ (30 mmol kg −1 ). Math1 deletion, followed by Notch inhibition, was performed by first injecting mice with β-naphthoflavone on day 0, followed by DBZ on day 14. All mice with double treatment were killed for analysis on day 21. Tissue sample preparation Freshly isolated intestines were flushed with formalin (4% formaldehyde in phosphate-buffered saline (PBS)) and fixed by incubation overnight in a 10-fold excess of formalin at room temperature. The formalin was removed and the intestines washed twice in PBS at room temperature. The intestines were then transferred to a tissue cassette and dehydrated by serial immersion in 20-fold volumes of 70, 96 and 100% EtOH for 2 h each at 4 °C. Excess ethanol was removed by incubation in xylene for 1.5 h at room temperature and cassettes were then immersed in liquid paraffin (56 °C) overnight. Paraffin blocks were prepared using standard methods. Immunohistochemistry and in situ hybridization Tissue sections of 4 μm thickness were de-waxed by immersion in xylene (two times, 5 min) and hydrated by serial immersion in 100% EtOH (two times 1 min), 96% EtOH (two times 1 min), 70% EtOH (two times 1 min) and distilled water (two times 1 min). Endogenous peroxidase activity was blocked by immersing the slides in peroxidase-blocking buffer (0.040 M citric acid, 0.121 M disodium hydrogen phosphate, 0.030 M sodium azide, 1.5% hydrogen peroxide) for 15 min at room temperature. Antigen retrieval was performed (see details below for each antibody), and blocking buffer (1% bovine serum albumin in PBS) was added to the slides for 30 min at room temperature. Primary antibodies were then added and incubated as detailed below. The slides were then rinsed in PBS and secondary antibody was added (polymer horseradish peroxidase-labelled anti-mouse/rabbit, Envision) for 30 min at room temperature. Slides were again washed in PBS and bound peroxidase was detected by adding diaminobuteric acid (DAB) substrate for 10 min at room temperature. Slides were then washed two times in PBS and nuclei were counterstained with Mayer's haematoxylin for 2 min, followed by two rinses in distilled water. Sections were dehydrated by serial immersion for 1 min each in 50% EtOH and 60% EtOH, followed by 2 min each in 70% EtOH, 96% EtOH, 100% EtOH and xylene. Slides were mounted in Pertex mounting medium and a coverslip was placed over the tissue section. Antigen retrieval was performed by boiling samples for 20 min in 10 mM sodium citrate buffer pH 6.0. Antibodies used were mouse anti-Ki67 (1:100 dilution; Novocastra), rabbit anti-Math1 (1:50 dilution), rabbit anti-synaptophysin (1:200 dilution; Dako), rabbit anti-lysozyme (1:1,750 dilution; Dako) and rabbit anti-Hes1 (1:150 dilution; Santa Cruz). Antibodies were incubated overnight in bovine serum albumin in PBS at 4 °C for antibodies directed against Math1, and for 1 h at room temperature for antibodies directed against Ki67, synaptophysin and lysozyme. In all cases, the Envision + kit (Dako) was used as a secondary reagent. Stainings were developed with DAB. Slides were counterstained with haematoxylin and mounted. For in situ hybridization, 8 μm-thick sections were rehydrated as described above. Thereafter, sections were treated with 0.2 M sodium chloride and proteinase K. Slides were post-fixed, and sections were then demethylated with acetic anhydride and prehybridized. Hybridization was carried out in a humid chamber with 500 ng ml −1 of freshly prepared digoxigenin-labelled RNA probe of Olfm4 (image clone 1078130). Sections were incubated for at least 48 h at 68 °C. The slides were washed and incubation of the secondary anti-digoxigenin antibody (Roche) was carried out at 4 °C overnight. The next day, sections were washed and developed using Nitro Blue Tetrazolium Chloride/5-Brom-4-Chlor-3-Indolyl-Phosphat. How to cite this article: van Es, J.H. et al . Intestinal stem cells lacking the Math1 tumour suppressor are refractory to Notch inhibitors. Nat. Commun. 1:18 doi: 10.1038/1017 (2010).